Regulation of the NaV1.5 cytoplasmic domain by calmodulin Voltage-gated sodium channels (Na v ) underlie the rapid upstroke of action potentials in excitable tissues. Binding of channel-interactive proteins is essential for controlling fast and long-term inactivation. In the structure of the complex of the carboxy-terminal portion of Na v 1.5 (CTNa v 1.5) with calmodulin (CaM)–Mg 2+ reported here, both CaM lobes interact with the CTNa v 1.5. On the basis of the differences between this structure and that of an inactivated complex, we propose that the structure reported here represents a non-inactivated state of the CTNa v , that is, the state that is poised for activation. Electrophysiological characterization of mutants further supports the importance of the interactions identified in the structure. Isothermal titration calorimetry experiments show that CaM binds to CTNa v 1.5 with high affinity. The results of this study provide unique insights into the physiological activation and the pathophysiology of Na v channels. Voltage-gated sodium channels (Na v ) are transmembrane glycoproteins that underlie the rapid upstroke of action potentials in excitable tissues such as the heart, skeletal muscle and brain. Mendelian-inherited mutations in Na v channels result in diseases of excitability such as myotonias, paralyses, cardiac arrhythmias and ataxias and seizure disorders [1] . Na channels consist of an α subunit and one or more β subunits, but only the pore-forming α subunit is essential for function. Ten different isoforms of mammalian α subunits (Na v 1.1–1.9, and Na x ) have been described, with different properties and tissue distribution. The transmembrane portion of the α subunit is formed by four homologous domains (DI–DIV), each containing six membrane-spanning helices (S1–S6) that form the ion-selective pore and contain the activation voltage sensors. Channel activation and opening is followed by prompt closure via a number of kinetically distinct inactivation states [2] . Fast inactivation (recovery τ <10 ms), the best characterized of these processes, involves occlusion of the cytoplasmic mouth of the channel by the interdomain DIII–DIV linker (DIII/IV). A triplet of hydrophobic residues of the linker, Ile-Phe-Met, is key for this inactivation [3] . Na V channels are regulated by the interaction of their carboxyl terminal (CT) domain, located in the cytoplasm of responsive cells, with various channel-interactive proteins [4] , [5] . The importance of these interactions is highlighted by the effects of mutations in the Na v CT domain (CTNa v ) on channel function: gain-of-function mutations of the Na V 1.5 CT domain (CTNa v 1.5) cause long QT syndrome and loss-of-function mutations result in Brugada syndrome. The proximal portion of the CTNa v (residues 1,776–1,929 in Na v 1.5) is comprised of six α-helices (αI–αVI) [6] , [7] . The first four helices αI–αIV, form an EF-hand-like motif (EFL) that has a fold similar to that of a the Ca 2+ -binding EF hand [8] , [9] , [10] . The fifth helix (αV) and a flexible loop connect the EFL to a long sixth helix (αVI), which contains an IQ motif that binds calmodulin (CaM) [7] . Several structural studies have explored the interaction of CaM with different regions of Na v channels. One structure, the complex of the C-lobe of CaM with the DIII/IV linker of Na V channels, suggests that CaM modulates fast inactivation by forming a bridge between the CTNa v IQ motif and the DIII/IV linker of the channel [11] , [12] . In the structure of the ternary complex containing CTNa V 1.5, apo-CaM and a fibroblast growth factor (FGF) homologous factor (FHF)—a long-term inactivator of Na v channels—FHF binds to the EFL of Na v 1.5 and the C-lobe of CaM binds to the IQ motif [7] . Together, these structural data point to complex dynamic interactions among the participating components in regulating channel gating. Despite the availability of biochemical, electrophysiological, biophysical and structural information, the participation of the CTNa v in the regulation of Na V channels is still a matter of debate and may be isoform-specific [8] , [13] , [14] . Given the central importance of Na V 1 channels, it is surprising that important details of the molecular mechanisms leading to their activation, inactivation and recovery from inactivation remain unknown. Missing, for example, are structures involving the cytoplasmic domain of Na v 1.5 when the channel is poised for opening. Here we present the structure of the complex of the C-terminal domain of the Na v 1.5 channel with CaM–Mg 2 + , which we propose, represents the resting state of the cytoplasmic region of the channel after the recovery from inactivation, that is, the state in which the channel is poised for activation. We will refer to this state as ‘non-inactivated’ or resting. Site-specific mutations at the sites of interactions identified in the structure presented here alter the inactivation properties of Na v 1.5, as determined by electrophysiological recordings. Calorimetric measurements show that CTNa v 1.5 binds tightly to full-length CaM, while the DIII–IV linker peptide cannot compete CTNa v 1.5 from the CTNa v 1.5–CaM complex. The results of this study provide unique insights into the physiological activation and the pathophysiology of Na v channels [15] . Overall structure of the CTNa v 1.5–CaM complex The crystal of the CTNa v 1.5–CaM–Mg 2+ complex (see below) determined to 2.8 Å contains five highly similar heterodimers in the asymmetric unit (ASU) (average r.m.s.d. 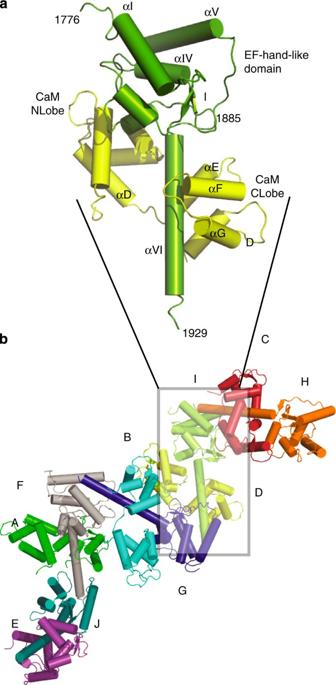Figure 1: CTNav1.5–CaM complex. (a) CTNav1.5–CaM complex with CTNav1.5 in lime-green and CaM in yellow. The helices of CTNav1.5 are labelled αI–VI and CaM helices αA–G. (b) The five CTNav1.5–CaM complexes in the asymmetric unit. The CaM molecules are labelled A, B, C, D, and E; the CTNav1.5 are labelled F, G, H, I, J. For example, AF is the heterodimer with CaM molecule A and CTNav1.5 molecule F. 1.6 Å), each composed of a full-length CaM (residues 1–148) and one CTNa v 1.5 (residues 1,776–1,929) ( Table 1 ; Fig. 1 ; Supplementary Table 1 ). Table 1 Data collection and refinement statistics. Full size table Figure 1: CTNa v 1.5–CaM complex. ( a ) CTNa v 1.5–CaM complex with CTNa v 1.5 in lime-green and CaM in yellow. The helices of CTNa v 1.5 are labelled αI–VI and CaM helices αA–G. ( b ) The five CTNa v 1.5–CaM complexes in the asymmetric unit. The CaM molecules are labelled A, B, C, D, and E; the CTNa v 1.5 are labelled F, G, H, I, J. For example, AF is the heterodimer with CaM molecule A and CTNa v 1.5 molecule F. Full size image In each heterodimer the CTNa v 1.5 has a bipartite structure resembling a lollipop ( Fig. 1a ) in which the globular EFL domain (residues 1,776–1,866), the head, is connected via helix αV (residues 1,866–1,884) and a loop (residues 1,885–1,894) to the long stalk (helix αVI; residues 1,895–1,929) ( Fig. 1a ). The structure of the EFL domain (helices αI–αIV; Fig. 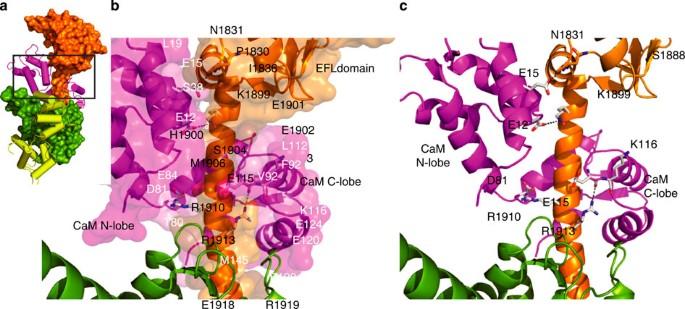Figure 2: Interaction of CTNav1.5 with CaM. (a) Overview of the heterodimer. (b) Surface representation of the residues involved at the interface of CTNav1.5 (orange) and the N- and C-lobe of CaM (magenta). The neighbouring CTNav1.5 is shown in green. (c) Hydrogen-bonding residues flanking the end of the interface (Glu12-Lys1899; Glu15-Asn1831; Glu115-Arg1913; Asp81-Arg1910). 1 ) is similar to the nuclear magnetic resonance structures of the EFL domains of Na v 1.5 (residues 1,773–1,865, protein data bank (PDB) id 2KBI, Supplementary Table 2 ) [16] and Na v 1.2 (PDB id 2KAV) [17] . CaM conformation in the Na v 1.5–CaM–Mg 2+ complex The CaM N-lobe (residues 1–77; helices αA–αD; Supplementary Fig. 1 ) adopts a ‘closed’ conformation and the C-lobe (residues 82–148; helices αE–αH) a ‘semi-open’ conformation ( Supplementary Fig. 1 ; Supplementary Fig. 2 ) [18] , [19] , [20] . A short linker (residues 78–81) connects the two lobes in such a way that the long axis of helix αD of the N-lobe (residues 65–77) is orthogonal to the αE helix of the C-lobe (residues 82–93) forming a ‘lock-washer’ type arrangement around helix αVI of the CTNa v 1.5 ( Fig. 1a ). This conformation of CaM is highly different from the one observed in the structure of the CTNa v 1.5–CaM-FGF13 (ref. 7 ) complex (PDB id 4DCK; FGF13=FHF2) in which helix αD, the linker and helix αE form a long nine-turn helix (residues 64–95) that places the CaM N-lobe at a significant distance from the CTNa v 1.5. Ion binding in the Na v 1.5–CaM–Mg 2+ complex Both CaM lobes of all five CaMs in the ASU contain bound ions. The lack of anomalous scattering signal at Cu Kα, a wavelength at which Ca 2+ and Mn 2+ have significant anomalous signal, and the observed coordination suggest that the ions are Mg 2+ from the crystallization solution [19] ( Supplementary Fig. 1 ). Significantly, the conformation of the N-lobe of CaM in the Na v 1.5–CaM–Mg 2+ complex reported here is highly similar to that of N-lobe of apo-CaM (PDB id 1DMO [18] ; Supplementary Fig. 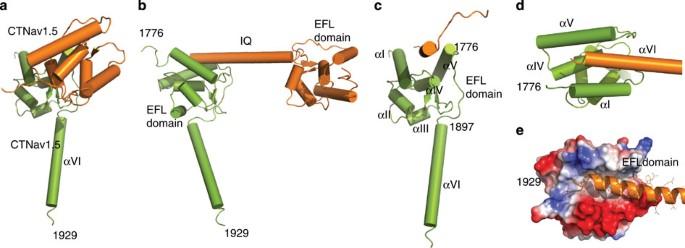Figure 3: Interaction of the CTNav1.5 EFL domain with a neighbouring CTNav1.5 helix αVI. (a) Front view of the CTNav1.5–CTNav1.5 dimer. Residues of one CTNav1.5 molecule (green) interact with another CTNav1.5 molecule (orange). (b) Same asabut rotated 90° fromain the plane of the figure. (c) 90° rotation frombshowing the concave cavity formed by the helices of the EFL domain; helix αI 1,788–1,801; helix αII 1,814–1,820; helix αIII 1,832–1,837; helix αIV 1,850–1,858; helix αV 1,866–1,882; helix αVI 1,897–1,926. (d) Close-up of the cavity formed by helices αI and αV with helix αVI. (e) Same asd, but with one CTNav1.5 coloured according to the electrostatic potential. It displays a hydrophobic surface with ionic patches at the beginning and end. 1 ) as well as to the N-lobe of the CaM–Mg 2+ complex (PDB id 3UCW; Supplementary Table 3 (ref. 19 )). In contrast, it is significantly different from that of the Ca 2+ -loaded CaM (PDB id 1CDM [21] ). The C-lobe of CaM in the Na v 1.5–CaM–Mg 2+ complex has the semi-open conformation observed in CaM structures such as that of the Na v 1.2-IQ–CaM complex, in which the cation-binding sites are not occupied by Ca 2+ (PDB id 2KXW; PDB id 3WFN, Supplementary Fig. 2 ) [22] , [23] . No ions are bound to the CTNa v 1.5 EFL domain in the CTNa v 1.5–CaM–Mg 2+ complex. This domain does not show density at the expected ion positions (‘Ca +2 -binding loops’; residues 1,802–1,812 and residues 1,838–1,850), and crucial acidic residues such as Glu1804 and Glu1846 are not in the conformations required for Ca +2 binding ( Supplementary Fig. 2 ). 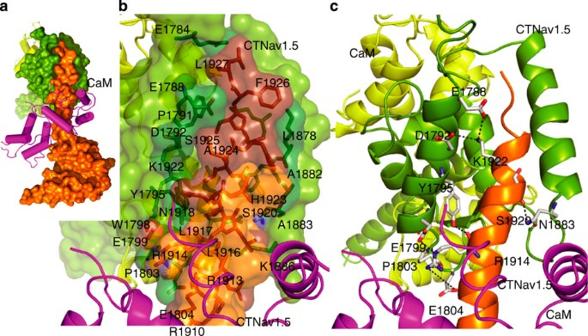Figure 4: Molecular view of the CTNav1.5 EFL domain with a neighbouring CTNav1.5 helix αVI. (a) Overview of the Nav1.5–Nav1.5 interaction. (b) Surface representation of the residues involved at the interface of CTNav1.5 helix αVI (orange and brown) with the neighbouring CTNav1.5 EFL (green and forest green) displaying the involved amino acids as sticks. (c) Ribbon representation of the interface showing the amino acid at the hydrogen-bonding distance. Hydrogen-bonding pattern of CTNav1.5 EFL (green and forest green) with the CTNav1.5 (orange and brown). CTNa v 1.5–CaM interaction In the complex reported here, CaM wraps around the long helix of Na v 1.5 in such a way that the interface buries ~1,400 Å 2 ( Supplementary Table 4 ), ~950 Å 2 between the C-lobe of CaM and the CTNa v 1.5 IQ and ~450 Å 2 between of the N-lobe and the Na v 1.5 EFL domain. The CaM–CTNa V 1.5 interface is mostly hydrophobic (29 EFL hydrophobic interactions; Fig. 2a,b ), but it is flanked at both ends by hydrogen bonds between the two proteins (7 H-bonds: Lys1899–Glu12, and Asn1831–Glu15, at one end and Arg1910–Asp81, Arg1913–Glu121, Arg1913–Glu115, Arg1919–Glu124 and Glu1901–Lys95 at the other; Fig. 2c ). Figure 2: Interaction of CTNa v 1.5 with CaM. ( a ) Overview of the heterodimer. ( b ) Surface representation of the residues involved at the interface of CTNa v 1.5 (orange) and the N- and C-lobe of CaM (magenta). The neighbouring CTNa v 1.5 is shown in green. ( c ) Hydrogen-bonding residues flanking the end of the interface (Glu12-Lys1899; Glu15-Asn1831; Glu115-Arg1913; Asp81-Arg1910). Full size image Interaction of CTNa v 1.5 EFL domain and helix αVI In the crystal structure reported here, the EFL domains (1,776–1,882) of each CTNa v 1.5 molecule contacts the C-terminal portion of helix αVI (1,910–1,926) of another CTNa v 1.5 molecule ( Fig. 3 ). This CTNa v 1.5–CTNa v 1.5 interaction (buried area ~900 Å; complementarity index 0.55 (ref. 24 )) is also mainly hydrophobic. It is flanked at both ends by salt bridges (Glu1804–Arg1910, Glu1799–Arg1914 and Asp1792–Lys1922) and hydrogen bonds (Tyr1795–Arg1914 and Asn1883–Ser1920) ( Figs 3 and 4 ). A helix αVI–EFL interaction was postulated by Chazin et al. [16] , and measured by Glaaser [25] by transition-metal ion fluorescence resonance energy transfer, but it was interpreted as an intramolecular interaction and not as an interaction between two molecules. Figure 3: Interaction of the CTNa v 1.5 EFL domain with a neighbouring CTNa v 1.5 helix αVI. ( a ) Front view of the CTNa v 1.5–CTNa v 1.5 dimer. Residues of one CTNa v 1.5 molecule (green) interact with another CTNa v 1.5 molecule (orange). ( b ) Same as a but rotated 90° from a in the plane of the figure. ( c ) 90° rotation from b showing the concave cavity formed by the helices of the EFL domain; helix αI 1,788–1,801; helix αII 1,814–1,820; helix αIII 1,832–1,837; helix αIV 1,850–1,858; helix αV 1,866–1,882; helix αVI 1,897–1,926. ( d ) Close-up of the cavity formed by helices αI and αV with helix αVI. ( e ) Same as d , but with one CTNa v 1.5 coloured according to the electrostatic potential. It displays a hydrophobic surface with ionic patches at the beginning and end. Full size image Figure 4: Molecular view of the CTNa v 1.5 EFL domain with a neighbouring CTNa v 1.5 helix αVI. ( a ) Overview of the Na v 1.5–Na v 1.5 interaction. ( b ) Surface representation of the residues involved at the interface of CTNa v 1.5 helix αVI (orange and brown) with the neighbouring CTNa v 1.5 EFL (green and forest green) displaying the involved amino acids as sticks. ( c ) Ribbon representation of the interface showing the amino acid at the hydrogen-bonding distance. Hydrogen-bonding pattern of CTNa v 1.5 EFL (green and forest green) with the CTNa v 1.5 (orange and brown). Full size image Calorimetric analysis Isothermal titration calorimetry at 28 °C ( Fig. 5a ) shows that CTNa v 1.5 binds CaM in an exothermic reaction with K d s ranging from 46±33 to 105±15 nM depending on the buffer conditions. The lack of significant enthalpies of binding of the III–IV linker to the CTNa v 1.5–CaM complex argues against the competition between III–IV and the C-lobe of CaM ( Fig. 5b ). 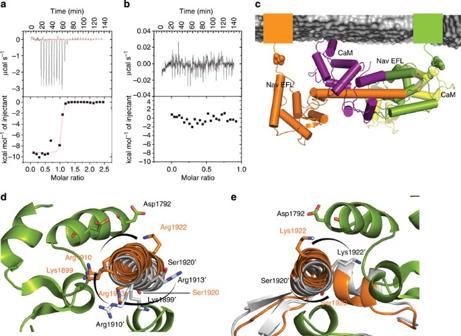Figure 5: Non-inactivated conformation of CTNav1.5–CaM. (a) Thermodynamic analysis of CTNav1.5 and CaM binding. Isotherms of CTNav1.5 titrated with CaM. Top panel displays the heat evolved following each injection and the bottom panel shows the integrated heats of injection. All the curves are fitted to a one-binding site per monomer model. (b) Thermodynamic analysis of CTNav1.5–CaM and III–IV linker binding. Isotherm of CTNav1.5–CaM titrated with the III–IV linker (residues 1,489–1,502). (panels as ina). Note the change in scale on theyaxis. (c) Attachment points of the N termini of the CTNav1.5 (coloured squares) to the transmembrane helices S6 of domain IV of the channel (not shown). (d) Overlap of CT helices αVI in the resting non-inactive conformation (orange) versus inactivated (grey). The rotation of the helix αVI is evidenced by the rotated positions of Lys1899, Arg1910, Arg1913 and Ser1920. This change highlights the disruption of the CTNav1.5–CTNav1.5 interaction caused by the rotation that results in the inactivated form of the channel. (e) Same asd, but seen from the C-terminal of helix αVI of the CTNav1.5. Figure 5: Non-inactivated conformation of CTNa v 1.5–CaM. ( a ) Thermodynamic analysis of CTNa v 1.5 and CaM binding. Isotherms of CTNa v 1.5 titrated with CaM. Top panel displays the heat evolved following each injection and the bottom panel shows the integrated heats of injection. All the curves are fitted to a one-binding site per monomer model. ( b ) Thermodynamic analysis of CTNa v 1.5–CaM and III–IV linker binding. Isotherm of CTNav1.5–CaM titrated with the III–IV linker (residues 1,489–1,502). (panels as in a ). Note the change in scale on the y axis. ( c ) Attachment points of the N termini of the CTNa v 1.5 (coloured squares) to the transmembrane helices S6 of domain IV of the channel (not shown). ( d ) Overlap of CT helices αVI in the resting non-inactive conformation (orange) versus inactivated (grey). The rotation of the helix αVI is evidenced by the rotated positions of Lys1899, Arg1910, Arg1913 and Ser1920. This change highlights the disruption of the CTNa v 1.5–CTNa v 1.5 interaction caused by the rotation that results in the inactivated form of the channel. ( e ) Same as d , but seen from the C-terminal of helix αVI of the CTNa v 1.5. Full size image Size-exclusion chromatography of CTNa v 1.5–CaM Size-exclusion chromatography (SEC) analysis shows that, in solution, CTNav1.5–CaM behaves as a heterodimer with a retention time corresponding to a complex with one molecule of CTNa v 1.5 and one of CaM ( Supplementary Fig. 3 ). The elution profile shows no indication of the presence of oligomers of this heterodimer. The most intriguing feature of the structure presented here is the presence of an intimate contact between the C-terminal portion of the Na v 1.5 helix αVI and the EFL domain of another Na v 1.5 molecule in an arrangement that can be described as an asymmetrical [CTNa v 1.5–CaM]–[CTNa v 1.5–CaM] homodimer ( Figs 1 , 3 and 4 ). This dimer may reflect the Na v 1.5–Na v 1.5 interaction reported in cells. Full-length Na v 1.5 was shown by co-immunoprecipitation to form homodimers when expressed in cells [26] , [27] . Moreover, this dimerization of Nav1.5 explains the effect of some dominant-negative disease-causing mutations. Although there is no direct evidence that the interface observed in the structure described here is part of this dimerization, there are other strong indications that the contact described in this manuscript is part of an important physiological interaction. First, all five Na v 1.5 monomers in the ASU participate in this exact same contact. The r.m.s.d. among the structures of the five heterodimers in the ASU range from 1.2 to 1.7 Å (for 270 Cα carbons aligned), indicating that this organization of two Na v 1.5 and two CaM molecules is conserved regardless of crystal contacts. Had these contacts only been present between molecules related by crystal symmetry, an argument could have been made that they are a consequence of crystal packing. That all molecules in the ASU make this contact points to a fundamental interaction. Second, this contact buries about 900 Å 2 with a complementarity index of 0.55 ( Supplementary Table 5 ). These values are more compatible with a true protein–protein interaction than with a crystal contact. Confirming this assessment, PISA [28] , the standard software for identifying protein–protein interactions, recognizes the interface between all complexes in the ASU, G and F, F and J, J and H, I and H and I and G [24] , as true dimers. Furthermore, residues that participate in this interface are well conserved among Na v isoforms ( Supplementary Fig. 4 ). Third, in the dimer, the N termini of the two CTNa v 1.5 monomers point in the same direction. This arrangement allows the N-terminal of both CTNa v 1.5 to simultaneously emerge as continuations of the helices S6 of their respective channels ( Fig. 5c ). In addition, in this arrangement, there are no clashes of any portion of the dimer of complexes (Na v 1.5–CaM) with the membrane ( Fig. 5c ). The functional (physiological) effect of this dimerization is discussed in the next section. The presence of a dimer of this construct is not detectable by SEC even at the highest concentrations achievable in solution ( Supplementary Fig. 3 ). This is not surprising. While the CTNa v 1.5 is connected to the rest of the channel it is constrained to a very small volume close to the cytoplasmic side of the membrane (two-dimensional case) resulting in a very high local concentration. In contrast, in solution the molecules are free to occupy any position in the bulk (three-dimensional case). This effect was discussed extensively before [29] , [30] , [31] . The case for dimerization of the cytoplasmic portion of Na v 1.5 is further strengthen by the observation that the full-length channel participates in functional dimers. The physiological relevance of the structure reported here can be recognized by comparing it with that of CTNa v 1.5 in complex with CaM and FHF2. FHF2 has been shown to promote long-term inactivation of Na v channels [5] , [32] , [33] . This observation can be construed as suggesting that binding of the FHF stabilizes an inactivated conformation of the channel by locking the complex of CTNa v 1.5 and CaM in a configuration that is not compatible with channel conductance. This conformation of the CTNa v 1.5–CaM portion of the complex shows large differences with the structure reported here. In the CTNa v 1.5–CaM-FGF13 (heterotrimer), CaM is in an extended conformation in which CaM helices αD–αE are fully extended, forming a single helix that includes the linker residues. The only interaction of CaM with the CTNa v 1.5 involves binding of the CaM C-lobe to the IQ motif. Because of the CaM extended conformation, the CaM N-lobe lies away from the CTNa v 1.5 in a position that would allow it to interact with the DIII–IV linker. In contrast, in the CTNa v 1.5–CaM structure, CaM is present in a conformation resembling a ‘lock-washer’ that allows its N-lobe to make significant contacts with the EFL domain of Na v 1.5 (area buried 450 Å 2 , Fig. 6 ). Although the interaction of the CaM C-lobe with the IQ of helix αVI is the same in both complexes, in the structure of the complex reported here, the relation between helix αVI and the EFL domain is markedly different: helix αVI is rotated by ~90° around its axis ( Fig. 5 ). Changes in the conformation of residues 1,892–1,895 of the Na v 1.5, which link the EFL domain to helix αVI, accommodate this rotation without significant changes in either the long helix or the rest of the EFL domain. This configuration of the Na v 1.5–CaM heterodimer is incompatible with the mode of binding of FGF13 in the tripartite inactivated complex. On the basis of these key differences, we propose that the structure reported here represents the non-inactivated (resting) state of the cytoplasmic portion of the Na v 1.5, that is, the configuration that is poised for opening of the channel. In this configuration, the heterodimer can form the asymmetric CTNa v 1.5–CaM/CTNa v 1.5–CaM homodimer described above. This dimerization stabilizes the non-inactivated conformation of the channel. 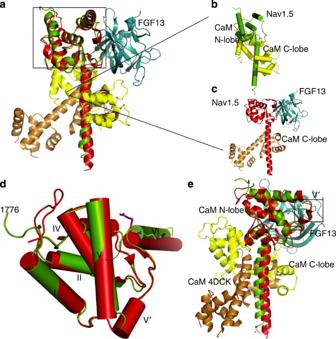Figure 6: Overlap of CTNav1.5–CaM with Nav1.5–CaM-FGF13 aligning their EFL domains. (a) CTNav1.5–CaM is shown in lime-green/yellow (this work; PDB 4OVN). (b) The alignment highlights the rotation of helix αVI by 90° with respect to the EFL domain. The CaM rotates with the helix. CTNav1.5–CaM is shown in lime-green/yellow (this work) and Nav1.5–CaM-FGF13 (PDB 4DCK, red; CaM, sand, FHF in cyan). (c) Nav1.5–CaM-FGF13 (PDB 4DCK). (d) Close-up of the EFL area boxed ina; Nav1.5–CaM-FGF13 has an extra helix V’. (e) Overlap of CTNav1.5–CaM with Nav1.5–CaM-FGF13 showing that the extended conformation of CaM is not conducive to the formation of a CTNav1.5–CTNav1.5 dimer; two residues in helix VI show the rotation of the helix. The residues shown are part of the charge–charge interaction of Nav1.5 IQ–CaM. Figure 6: Overlap of CTNa v 1.5–CaM with Na v 1.5–CaM-FGF13 aligning their EFL domains. ( a ) CTNa v 1.5–CaM is shown in lime-green/yellow (this work; PDB 4OVN). ( b ) The alignment highlights the rotation of helix αVI by 90° with respect to the EFL domain. The CaM rotates with the helix. CTNav1.5–CaM is shown in lime-green/yellow (this work) and Na v 1.5–CaM-FGF13 (PDB 4DCK, red; CaM, sand, FHF in cyan). ( c ) Nav1.5–CaM-FGF13 (PDB 4DCK). ( d ) Close-up of the EFL area boxed in a ; Na v 1.5–CaM-FGF13 has an extra helix V’. ( e ) Overlap of CTNa v 1.5–CaM with Na v 1.5–CaM-FGF13 showing that the extended conformation of CaM is not conducive to the formation of a CTNa v 1.5–CTNa v 1.5 dimer; two residues in helix VI show the rotation of the helix. The residues shown are part of the charge–charge interaction of Na v 1.5 IQ–CaM. Full size image In summary, the conformation of the CTNa v 1.5–CaM heterodimer appears to control the state of the channel. When in the conformation observed in the Na v 1.5–CaM-FGF13 complex the channel is inactivated—it cannot conduct. This conformation is stabilized by binding FHFs. In the structure reported here, the CaM N-lobe interacts with the Na v 1.5 EFL. As a result, the C-lobe changes its orientation with respect to the EFL by 90° and rotates with its helix αVI to the conformation that is ready for activation, that is, the non-inactivated state. This conformation is stabilized by the formation of the CaM–Na v 1.5–Na v 1.5–CaM homodimer. We propose that under physiological conditions, when the two CTNa v 1.5 that form the homodimer are connected to the rest of their channels, only one of the two channels becomes non-inactivated and ready to open. Activation through the formation of an asymmetric homodimer has been proposed for another membrane protein, the EGF tyrosine kinase receptor, also based on an interaction observed in the crystal structure of its cytoplasmic C-terminal domain [34] . All CaM molecules in the structure reported here contain Mg 2+ in their EF hands and therefore adopt the conformation observed in the structures of other CaM–Mg 2+ complexes and in the structures of apo-CaM. The arrangement of the CTNa v 1.5 and CaM in the homodimers is not compatible with the CaM conformation of the CaM–Ca 2+ complexes, indicating that the non-inactivated state can only be achieved with apo or Mg 2+ -bound CaM. Since the cellular concentration of Mg 2+ is maintained in the range 0.5–1.0 mM—that is, above the K d of CaM for Mg 2+ —CaM most likely binds Mg 2+ during the portion of the cycle when Ca 2+ is at its resting concentration. Thus, when the channel changes from inactivated to non-inactivated, Ca 2+ ions bound to the CaM EF hands are replaced by Mg 2+ , allowing the N-lobe to interact with the EFL domain and favouring formation of the Na v 1.5–Na v 1.5 homodimer. Using the available structures, many mutations observed in cardiac arrhythmias map to the interfaces of CTNa v 1.5 with channel-interactive proteins or other regions of the channel including the DIII–IV linker. For example, Q1909R, associated with LQT3, produces a substantial depolarizing shift in steady-state inactivation ( Fig. 7 ; Table 2 ). Another mutation Q1909A destabilizes CaM binding to the CTNa v 1.5 IQ domain in vitro ( Table 2 [13] ; Supplementary Fig. 5 ). In contrast, a mutation at the adjacent position, R1910A, has no significant effect on channel gating ( Table 2 ; Supplementary Fig. 5 ). 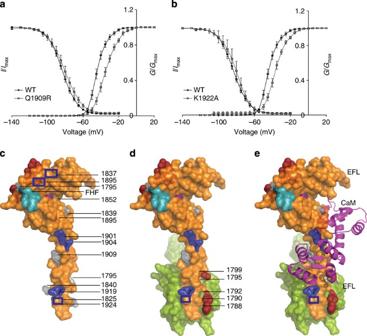Figure 7: Mutations affecting CTNav1.5–CaM and CTNav1.5–CTNav1.5 interactions. (a,b) Electrophysiological features of Na+channel variants altered at the CTNav1.5–CaM–Ca2+interaction interface. Activation and steady-state inactivation of wild-type (circles) and mutant channels (squares). The data are fit to a Boltzman function as described in Methods. Mutant channels and Q1909R and K1922A exhibit a depolarizing shift in theV0.5of inactivation (Supplementary Fig. 5). (c) Surface representation of one monomer (orange) interacting with a neighbouring molecule (lime green). CTNav1.5 with LQT3 mutations (1795, 1825, 1840, 1895, 1909 and 1924) shown in grey and brugada syndrome mutations in blue (1837, 1901, 1904 and 1919). Epilepsy mutations at the interface with the CaM-C-term lobe (1895 and 1852) are shown in purple; Brugada mutations (1901 and 1904) are at the interface of CTNav1.5 with the CaM-C-term lobe (blue) and 1705, 1825, 1840 and 1924 are at the CTNav1.5–CTNav1.5 interface. Residues 1788, 1790, 1792 and 1799, shown in dark red, line the EFL-binding site for helix αVI residues past the IQ motif14. Residues of the FGF13 that contact the EFL domain are coloured turquoise. (d) Same ascdisplaying the neighbouring CTNav1.5. (e) Same orientation as incandd, including CaM as a magenta ribbon. Figure 7: Mutations affecting CTNa v 1.5–CaM and CTNa v 1.5–CTNa v 1.5 interactions. ( a , b ) Electrophysiological features of Na + channel variants altered at the CTNa v 1.5–CaM–Ca 2+ interaction interface. Activation and steady-state inactivation of wild-type (circles) and mutant channels (squares). The data are fit to a Boltzman function as described in Methods. Mutant channels and Q1909R and K1922A exhibit a depolarizing shift in the V 0.5 of inactivation ( Supplementary Fig. 5 ). ( c ) Surface representation of one monomer (orange) interacting with a neighbouring molecule (lime green). CTNa v 1.5 with LQT3 mutations (1795, 1825, 1840, 1895, 1909 and 1924) shown in grey and brugada syndrome mutations in blue (1837, 1901, 1904 and 1919). Epilepsy mutations at the interface with the CaM-C-term lobe (1895 and 1852) are shown in purple; Brugada mutations (1901 and 1904) are at the interface of CTNa v 1.5 with the CaM-C-term lobe (blue) and 1705, 1825, 1840 and 1924 are at the CTNa v 1.5–CTNa v 1.5 interface. Residues 1788, 1790, 1792 and 1799, shown in dark red, line the EFL-binding site for helix αVI residues past the IQ motif [14] . Residues of the FGF13 that contact the EFL domain are coloured turquoise. ( d ) Same as c displaying the neighbouring CTNa v 1.5. ( e ) Same orientation as in c and d , including CaM as a magenta ribbon. Full size image Table 2 Effect of CTNa v 1.5 mutations on steady-state activation and inactivation. Full size table The physiological effects of many mutations in the CT were previously difficult to understand. Some of these can now be explained using the Na v 1.5–Na v 1.5 homodimer interface identified here ( Fig. 7 ). For example, the mutation of K1922A produces a depolarizing shift in steady-state inactivation. Interestingly, K1922 is involved in a salt bridge that links helix VI to EFL residue E1788 ( Figs 4 and 7 ). Rotation of helix αVI in the inactivated conformation disrupts this interaction ( Fig. 5d ). In contrast, mutations of R1914, which is part of the same interface, produce a smaller shift in gating ( Table 2 ; Supplementary Fig. 5 ). Residues 1,924 and 1,914, mutated in Brugada syndrome, are at the Na v 1.5–Na v 1.5 interaction interface. A1924T was predicted to be at the CaM–IQ motif interface [35] ; however, Chazin et al. [36] showed that this residue was not in contact with CaM but with the EFL domain and suggested that the alanine residue is in a dynamic region as a possible explanation. The structure of the CTNa v 1.5–CaM provides a direct explanation for the dysfunction: the intermolecular interaction of the Na v 1.5 helix αVI with the Na v 1.5 EFL domain of another channel ( Fig. 7 ), brings residue 1,924 in close proximity to residues Met1851 and Met1875 of the interacting CTNa v 1.5 ( Fig. 7 ). Other mutations that result in significant alterations in inactivation of gating include mutations in the Na V 1.5–Na V 1.5 interface that can only be explained by the structure reported here. Notably, mutations in the αI helix of the EFL (for example, D1790G and E1788A/D1790A/D1792A/E1799A) markedly shift the steady-state inactivation ( V 0.5 ) in the hyperpolarizing direction and result in slow recovery from inactivation ( Table 2 ). Direct binding measurements provided additional information about binding among cytoplasmic components. On the basis of isothermal titration calorimetry (ITC) experiments, Sarhan et al . [12] suggested that the DIII–IV linker of Na v 1.5 (residues 1,489–1,522) binds the C-lobe of CaM ( K d ≈19 μM) and that this is the sole anchor point of binding of the DIII–IV peptide. In the structure reported here, however, the IQ portion of the helix αVI of Na v 1.5 binds to the same region of CaM as the DIII–IV linker, but in the opposite orientation ( Supplementary Fig. 6 ). In solution, CTNav1.5 binds CaM with high affinity ( K d ≈50 nM). The ITC titration of the CTNa v 1.5–CaM complex with the DIII–IV linker peptide (see Methods) does not show significant enthalpy of binding, suggesting that the DIII–IV linker may not be able to displace the IQ from CaM binding ( Fig. 5b ). This result suggests that after a dimerized channel opens a change takes place in the Na v 1.5–Na v 1.5 interaction that releases one of the two lobes of CaM for fast inactivation by DIII–IV binding ( Fig. 8 ). We propose that as part of this change, it is the N-lobe of CaM that is released from its interaction with the EFL and binds the DIII/IV of the same channel. In addition, we also propose that the C-lobe of CaM remains bound to the IQ and that the linker between the two CaM lobes adopts the extended helical configuration observed in the Na v 1.5–CaM–FHF structure. This arrangement would set up Na v 1.5 for binding FHF for long-term inactivation. A schematic representation of the relevant states is shown in Fig. 8 . An important question can be asked: How does the increase in the intracellular Ca 2+ concentration affect these states? One possible explanation is that Ca 2+ ions will bind to CaM and change its conformation, including the conformation of both lobes. These changes would have a significant impact on the way that CaM interacts with the CTNav1.5 and as a result, on the regulation of channel activation. 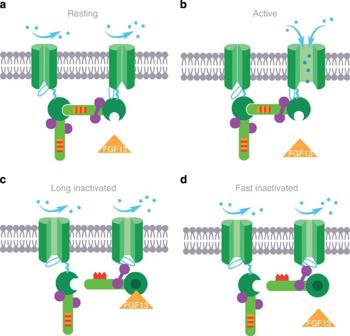Figure 8: Proposed mechanism of Nav1.5 regulation by the Nav1.5 cytoplasmic domain. Nav1.5 is coloured in green with a serrated marker in helix αVI to highlight the 90° rotation. Calmodulin is shown in purple. (a) Resting state showing the intermolecular interaction of the Nav1.5 poised for activation. (b) Active. N-lobe of CaM interacts with the EFL domain of Nav1.5; C-lobe of CaM interacts with IQ of helix αVI. (c) Long inactivated. FGF13 bound to the EFHL. (d) Fast inactivated. N-lobe of CaM releases the EFL-like and possible interacts with the III–IV linker. Helix αVI rotates 90°. Figure 8: Proposed mechanism of Na v 1.5 regulation by the Na v 1.5 cytoplasmic domain. Na v 1.5 is coloured in green with a serrated marker in helix αVI to highlight the 90° rotation. Calmodulin is shown in purple. ( a ) Resting state showing the intermolecular interaction of the Na v 1.5 poised for activation. ( b ) Active. N-lobe of CaM interacts with the EFL domain of Nav1.5; C-lobe of CaM interacts with IQ of helix αVI. ( c ) Long inactivated. FGF13 bound to the EFHL. ( d ) Fast inactivated. N-lobe of CaM releases the EFL-like and possible interacts with the III–IV linker. Helix αVI rotates 90°. Full size image The intricate set of interactions observed in the structure of the complex presented here, that includes binding of both CaM lobes to the CTNa v 1.5, as well as an apparent asymmetric dimerization of two Na v 1.5s, suggests a basis for an exquisite mechanism for switching from the inactivated to the non-inactivated form of the Na v 1.5 channel ( Fig. 8 ). This model also provides a rationale for disease-causing mutations that until now have escaped explanation. Cloning Complementary DNA (cDNA) corresponding to amino acids 1,773–1,929 of the Homo sapiens Na v 1.5 sodium channel α-subunit (CTNa v 1.5) was cloned into the pGEX-6-P1 vector. The entire H. sapiens CaM gene was cloned into the pET24b vector using the BamHI and NdeI sites. Expression and purification of the CTNa v 1.5–CaM complex B834 (DE3) methionine auxotroph cells were transformed with both the CTNa v 1.5-containing and CaM-containing plasmids simultaneously. The cells were grown overnight at 37 °C in 50 ml of LB medium supplemented with 50 μg ml −1 kanamycin and 100 μg ml ampicillin. The overnight culture was centrifuged, the LB media was discarded and the cells were resuspended in 50 ml of 1 × M9 media containing 50 μg ml kanamycin and 100 μg ml −1 ampicillin. Ten ml of the resuspension was used to inoculate 1 l of M9 media containing 0.05 mg ml −1 selenomethionine, 50 μg ml −1 kanamycin, 100 μg ml −1 ampicillin and additives as described by Leahy et al. [37] The cells were grown at 37 °C to an absorbance of 0.6 and protein expression was induced with 0.1 mM isopropyl β- D -1-thiogalactopyranoside. The cells were grown for an additional 5 h, centrifuged and the pellet was frozen at −80 °C. After thawing, pellets were resuspended in 40 ml 1 × phosphate-buffered saline (PBS) with a mixture of protease inhibitors: 2 μg ml −1 pepstatin A, 50 μg ml −1 leupeptin and 35 μg ml −1 phenylmethanesulfonyl fluoride (PMSF) per liter of culture. An additional 40 ml of 1 × PBS containing 2 mg ml −1 lysozyme were added, along with Triton X-100 to bring the final detergent concentration to 1%. The solution was incubated at 4 °C for 1.5 h with shaking, sonicated on ice in 15 s bursts for a total of 1 min and spun at 15,000 r.p.m. for 30 min. The supernatant was filtered through a 0.22 μm polyethersulfone (PES) filter, and loaded on a 25 ml Glutathione Sepharose 4 Fast Flow resin using a hydrostatic pump at 0.5 ml min −1 . The column was washed with 1 × PBS at 1 ml min −1 for a total of six resin volumes and protein was eluted in aliquots of 15 ml with an elution buffer containing 154 mg of reduced L-glutathione in 50 mM Tris-HCl at pH 8. Protein concentration in the samples was measured using a Nanodrop, and purity was assessed on a 4–12% Bis-Tris gel stained using Coomasie blue. Samples were stored on ice overnight at 4 °C. Prescission protease (0.3 mg) was added to the GST-CTNav1.5–CaM complex per 10 mg of protein. The protein was dialysed overnight against 50 mM Tris pH 7.0, 1 mM dithiothreitol. The next day, the protein was loaded onto a Source Q column. The eluate from the Source Q column was concentrated to 55 mg ml −1 and stored at −80 °C. Purity was assessed at each step by SDS–polyacrylamide gel electrophoresis. Visual inspection revealed a purity of at least 95%. Structure determination The CTNa v 1.5–CaM wild-type and selenomethionine-derivatized protein complex were crystallized by hanging-drop vapour diffusion at 18 °C by 1.2 :0.8 ratio of protein at 35–55 mg ml −1 and a well solution containing 15% polyethylene glycol 4K, 0.2 M MgSO 4 and 10% glycerol. Prior to data collection, crystals were transferred to the reservoir solution supplemented with additional glycerol and flash-frozen in liquid nitrogen. Data for native protein crystals were collected at the home source; multiwavelength anomalous diffraction (MAD) data for the selenomethionine-derivatized crystals were collected at APS on the LRL-CAT beamline 31A and at the National Synchrotron Light Source beamline X6A at the Se peak wavelength of 0.97989 Å. Indexing and data reduction were carried out with HKL2000 (ref. 38 ). The crystal contained five CTNav1.5–CaM complexes in the ASU. Phases were determined with SHARP [39] using data from the SeMet crystal. The positions of 47 out of the 90 seleniums atoms (8 methionine residues in CTNa v 1.5, 10 methionine residues in CaM with 5 heterodimers in the ASU) were determined by the program followed by phase determination, map calculation, density modification and initial model building to 3.3 Å. Non-crystallographic symmetry averaging with the Solomon (density modification) program of the AutoSharp suite [40] was used to extend the phases to 3.0 Å using a solvent content of 55%. The map generated using these improved phases allowed a combination of automatic and manual tracing of the protein backbone followed by iterative cycles of manual model building with Coot [41] and refinement with Refmac5 in the CCP4i suite. [40] The model of the SeMet-derivatized protein was used as a molecular replacement search model [42] for the native protein, which diffracted to a higher resolution. Model building was completed with iterative cycles of manual model building with Coot and refinement with Refmac5 (ref. 40 ). The correctness of the alignment of the sequence to the electron density was ascertained using the selenomethionine sites determined in SHARP. The final model was refined to 2.8 Å with R work and R free values of 21.6 and 28.3, respectively ( Supplementary Table 1 ). The quality of the structure was validated with Procheck [43] and Molprobity [44] . Residues (82.6%) are in the favoured region of the Ramachandran plot, 14.9% in additional allowed region and no residues in the disallowed region. The final model contains a total of 1352 amino acids. Buried surface areas were calculated using Protein Interfaces, Surfaces, and Assemblies (PISA) software [24] . Native data collected at Cu Kα was used to calculate anomalous maps to verify the absence of Ca 2+ bound to CTNa v 1.5–CaM–Mg 2+ . Size-exclusion chromatography Gel filtration of 200 μl CTNa v 1.5–CaM 40 mg ml −1 was performed ( n =5) on a Superdex 75 10/300 GL column on an AKTA FPLC (GE Lifesciences) in 50 mM Tris Cl pH 7.0, 150 mM NaCl, 1 mM dithiothreitol with and without 20 mM MgSO 4 . The protein standards albumin (66 kDa) and carbonic anhydrase (29 kDa) were used to calibrate the column. Isothermal calorimetry ITC experiments were performed with CTNa v 1.5 75 μM and 1 mM CaM. The protein in the sample cell was titrated with 25 10 μl injections of CaM. ITC experiments were performed with CTNa v 1.5–CaM and III–IV peptide (residues 1,489–1,502). The protein complex was diluted to a concentration of 40 μM (in monomers) in a buffer containing 10 mM Na 2 HPO 4 , 2 mM KH 2 PO 4 , 2.7 mM KCl, 137 mM NaCl, pH 7.4. The III–IV peptide was prepared in the same buffer at a concentration of 0.5 mM. Protein (1.8 ml) in the sample cell was titrated with twenty-five 10-μl injections. The data were analysed with Origin-5.0 software and fitted to a single binding site per monomer. Cellular electrophysiology The Na V 1.5 mutations were made by site-directed mutagenesis of Na V 1.5-GFP cDNAs using the Strategene Quickchange XL kit [14] . Approximately 0.75 × 10 6 human embryonic kidney cells (HEK293; American Type Culture Collection, Manassas, VA) were cultured in six-well tissue culture dishes in Dulbecco's modified Eagle's medium supplemented with foetal bovine serum 10%, L-glutamine (2 mmol l −1 ). The cells were co-transfected with plasmids encoding the appropriate Na V 1.5-GFP and Na V β1 subunit cDNAs as previously described [14] . Cells were transfected using Lipofectamine 2000 (Invitrogen) according to the manufacturer’s instructions and were studied at 48 h post transfection. The total amount of DNA for all transfections was kept constant. Whole-cell I Na was measured under voltage-clamp with an Axopatch 200B patch-clamp amplifier (Molecular Devices Corp.) at room temperature (22 °C). Voltage command protocols were generated by custom-written software and PCLAMP 10. Capacitance compensation was optimized and series resistance was compensated by 40–80%. Membrane currents were filtered at 5 kHz and digitized with 12-bit resolution through a DigiData-1200 interface (Molecular Devices Corp.). The patch pipettes had 1–2 MΩ tip resistances when filled with a pipette solution containing: 10 mM NaF, 20 mM CsCl, 100 mM CsF, 10 mM HEPES, 5 mM BAPTA, 4 mM CaCl2, pH 7.3 with CsOH. The bath solution contained 145 mM NaCl, 4 mM KCl, 1.8 mM CaCl 2 , 1 mM MgCl 2 , 10 mM glucose, 10 mM HEPES (pH 7.4 with NaOH). Standard voltage-clamp protocols were used to characterize the voltage dependence of activation and inactivation and recovery from inactivation. To determine the V 1/2 and slope factor k, steady-state inactivation data were fit with a Boltzmann function of the form: I / I max ={1+exp[(V−V 1/2 )/k]} −1 . Recovery from inactivation data were fit with a bi-exponential function of the form: using a nonlinear least squares minimization. Accession codes: Coordinates and structure factors have been deposited in the Protein Data Bank with accession code 4OVN . How to cite this article: Gabelli, S. B. et al. Regulation of the Na V 1.5 cytoplasmic domain by calmodulin. Nat. Commun. 5:5126 doi: 10.1038/ncomms6126 (2014).